Improving palm oil quality through identification and mapping of the lipase gene causing oil deterioration The oil palm fruit mesocarp contains high lipase activity that increases free fatty acids and necessitates post-harvest inactivation by heat treatment of fruit bunches. Even before heat treatment the mesocarp lipase activity causes consequential oil losses and requires costly measures to limit free fatty acids quantities. Here we demonstrate that elite low-lipase lines yield oil with substantially less free fatty acids than standard genotypes, allowing more flexibility for post-harvest fruit processing and extended ripening for increased yields. We identify the lipase and its gene cosegregates with the low-/high-lipase trait, providing breeders a marker to rapidly identify potent elite genitors and introgress the trait into major cultivars. Overall, economic gains brought by wide adoption of this material could represent up to one billion dollars per year. Expected benefits concern all planters but are likely to be highest for African smallholders who would be more able to produce oil that meets international quality standards. Oil extracted from the oil palm ( Elaeis guineensis ) [1] fruit mesocarp is the largest source of vegetable oil, with a world market share of ~32% ( Fig. 1a ). The share of palm oil production by small, family-owned, estates is 30% worldwide and reaches 80% in Nigeria, Africa’s largest producer [2] . It is expected that the oil palm share of the market will need to increase to meet the doubled demand for vegetable oil predicted by 2030 (refs 3 , 4 , 5 , 6 ). One major constraint that weighs heavily on yield and harvest management is the rapid oil acidification due to the high lipase (HL) activity that releases free fatty acids (FFA) in the mesocarp of bruised ripe fruits [7] , [8] , [9] , [10] . Acidity has a strong impact on the quality of commodity oil because an FFA content of >5% is considered to be unfit for human consumption [11] . 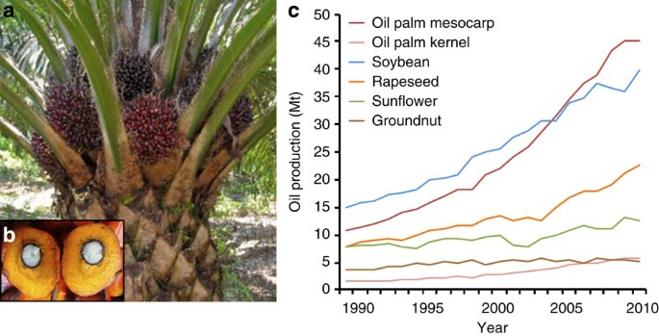Figure 1: Oil palm is a major oil-crop. (a) Palm tree with several bunches at different stages of ripeness; a palm tree continuously produces bunches yearlong (8–28 bunches per year, depending on age). While most cultivated trees are derived from Deli germplasm, several other germplasms such as La Me are significantly used by breeders. (b) Opentenerafruits showing fleshy mesocarp from which palm oil is extracted and kernel that contains an oil with shorter fatty acids. The amount of mesocarp per fruit is heavily influenced by the Sh gene that governs shell thickness.Teneratrees, which are the most productive and most widely cultivated, are heterozygous Sh+/−. Dura trees are Sh+/+ and contain a thicker shell and a thinner mesocarp, thus producing less oil. (c) World vegetable oil production by crop, showing the increasing share of palm oil (FAOSTAT,http://faostat.org, Dec 2011). Figure 1: Oil palm is a major oil-crop. ( a ) Palm tree with several bunches at different stages of ripeness; a palm tree continuously produces bunches yearlong (8–28 bunches per year, depending on age). While most cultivated trees are derived from Deli germplasm, several other germplasms such as La Me are significantly used by breeders. ( b ) Open tenera fruits showing fleshy mesocarp from which palm oil is extracted and kernel that contains an oil with shorter fatty acids. The amount of mesocarp per fruit is heavily influenced by the Sh gene that governs shell thickness. Tenera trees, which are the most productive and most widely cultivated, are heterozygous Sh+/−. Dura trees are Sh+/+ and contain a thicker shell and a thinner mesocarp, thus producing less oil. ( c ) World vegetable oil production by crop, showing the increasing share of palm oil (FAOSTAT, http://faostat.org , Dec 2011). Full size image Lipase activity can hydrolyze 30% of the oil content within 5 min [10] and large-scale exploitation of oil palm became feasible only after Fickendey [12] found a century ago that the lipase could be inactivated by heat treatment of harvested bunches. However, the mesocarp lipase can be active prior to heat treatment and release FFA. While FFA level of crude palm oil from large estates is usually 3–4% [13] , oil from smallholders shows higher values especially in Africa where FFA level reaches 9% in Nigeria [14] and can exceed 15% [15] . FFAs have to be removed through an energy-costly refining process that leads to oil losses [13] , so that most of the palm oil produced by African smallholders is not competitive on international markets [14] . To limit acidity, the bunches must be harvested before they are overripe, heat-sterilized rapidly (ideally within 1 day) to inactivate lipase activity and processed immediately. However, bunches also need to be harvested when they are as ripe as possible to maximize oil yield. These conflicting requirements narrow the harvest window down to ~1 week and oblige planters to harvest every 7–10 days, as oil palm continuously produces fruit bunches yearlong ( Fig. 1a ). As a result, more than a third of the plantation-operating costs are dedicated to harvest [1] . Palm oil is currently the least expensive oil on the market, due to high productivity and low labour costs in the producing countries, mainly Indonesia and Malaysia [4] . This will most likely change in the future as oil palm harvest is largely non-mechanized and labour-intensive, and wages are steadily increasing as Southeast Asia develops [1] , [4] . It is therefore important that management improves to keep harvest-associated costs as low as possible. While oil acidification concerns all planters, it is more acute for smallholders who may not have access to efficient milling facilities close to their plantation and whose overripe bunches may be rejected by mills. Indeed, the problem extends from the whole industry down to the consumer in those African countries where crude, unrefined, palm oil is a major commodity oil. The economic importance of palm oil acidity made the mesocarp lipase the most widely studied enzyme of oil palm [16] , as early as in 1910 (ref. 12 ). However, the source of this lipase activity has not yet been identified. We previously identified trees with a low mesocarp lipase activity [11] . Here we show that the oil extracted from these trees, using different procedures that mimic standard processes, have significantly lower acidity than that from the standard, HL genotypes currently cultivated. We also demonstrate that the low-/high-acidity trait is monogenic and identify the lipase responsible for oil acidity. Finally, we show that the lipase gene cosegregates with the low (LL)/HL trait, making it a useful DNA marker for marker-assisted selection of the trait, a key technique for fast breeding of crop trees [17] . Oil FFA content is lower in LL lines To assess the performance of LL trees, we used either elite tenera material ( Fig. 1 ) from a Deli (D1) × La Mé (L1) cross already used for commercial oil production or progenies of its dura Deli (D1) parent. The oil extraction ratio was 22.15% to 21.73% in HL and LL lines from D1, respectively, thus showing no influence of the LL trait on oil yield ( Table 1 ). Table 1 Yield is not affected in low-lipase lines. Full size table When ripe bunches were heat-sterilized a few hours after harvest, the oil extracted from standard fruits contained 0.66±0.36% (s.d.) FFA, while the oil from LL fruits showed less than half FFA, down to 0.30±0.02% ( Fig. 2a ). These ideal conditions are rarely met in practice and the average acidity of crude palm oil from large estates is usually ~3–4% [13] and can exceed 10% in small plantations. Therefore, we further focused on two critical steps of fruit processing that increase oil acidity: delayed harvesting of bunches and post-harvest delayed processing. When bunches were left on trees up to 30 days after ripeness, the oil from standard trees contained >12% FFA, whereas that from LL trees showed only half that value ( Fig. 2b ). Therefore, it is clear from our data that the use of LL genotypes should allow significant extended ripening without a negative impact on oil quality. This should increase oil yield as oil content of the bunches increases by ~7% after first fruit drop starts [18] , [19] . 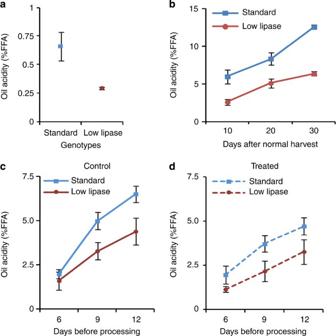Figure 2: LL genotype yields oil of lesser acidity than standard HL genotypes. (a) Ripe bunches (1–5 fallen fruits) were heat-sterilized a few hours after harvest. Oil was extracted immediately and its acidity titrated, expressed as %FFA).n=4 for LL fruits and 8 for HL (b) Overripe bunches were left up to 30 days on the tree after ripeness (1–5 fallen fruits) before harvest. Bunches and fallen fruits were then sterilized and processed. (c,d) Fruits were sprayed with water (control,c) or with fungicide (d), sun-dried and stored up to 12 days before heat sterilization and oil extraction;n=3–5. Analyses of variance were carried out according to the general linear model and differences between standard and LL materials were significant atP<0.001 (a–c) andP<0.012 (d) (Tukey’s test). Bunches were harvested from the segregating D1 × L1 cross (a,candd) or from selfed D1 progenies (LL P4 and standard P5, see plant material in Material and Methods section) (b). Error bars represent s.d. Figure 2: LL genotype yields oil of lesser acidity than standard HL genotypes. ( a ) Ripe bunches (1–5 fallen fruits) were heat-sterilized a few hours after harvest. Oil was extracted immediately and its acidity titrated, expressed as %FFA). n =4 for LL fruits and 8 for HL ( b ) Overripe bunches were left up to 30 days on the tree after ripeness (1–5 fallen fruits) before harvest. Bunches and fallen fruits were then sterilized and processed. ( c , d ) Fruits were sprayed with water (control, c ) or with fungicide ( d ), sun-dried and stored up to 12 days before heat sterilization and oil extraction; n =3–5. Analyses of variance were carried out according to the general linear model and differences between standard and LL materials were significant at P <0.001 ( a – c ) and P <0.012 ( d ) (Tukey’s test). Bunches were harvested from the segregating D1 × L1 cross ( a , c and d ) or from selfed D1 progenies (LL P4 and standard P5, see plant material in Material and Methods section) ( b ). Error bars represent s.d. Full size image Another critical step is the delay between harvest and bunch processing, especially in small estates distant from mills. When ripe bunches were processed 3 days after harvest, FFA content of oil from the standard genotype was 1.50±0.51% compared with only 0.35±0.09% from LL trees. The latter value is almost identical to that observed when bunches are processed immediately after harvest. When processing was further delayed, FFA content was still <5% at 12 days in LL lines ( Fig. 2c ). This result clearly indicates that LL lines will allow larger delays for processing bunches. This should strongly benefit smallholders distant from mills in areas lacking good transportation infrastructures [2] , as is frequently the case in Africa and for those who traditionally leave the bunches to ferment for several days before processing to allow fruit loosening [20] . There is a controversy as to the respective contributions of endogenous and fungal lipases to oil acidity [21] . Treating bunches with fungicide upon harvest ( Fig. 2d ) led to reduced oil acidity, with the oil from LL fruits containing 3% FFA after 12 days. Again, the oil from LL trees contained 30% less FFA compared to that of standard trees. Our data show that, although both mesocarp and fungal lipases are contributors to oil acidity, the endogenous lipase is clearly the dominant contributor to the immediate post-harvest rise in FFA. To conclude, in conditions known to favour high levels of FFA, LL genotypes always showed a delayed development of acidity when compared to the standard genotype. Therefore, clearly the LL genotypes can produce an oil of significantly lower acidity and therefore higher quality than that from presently used genotypes. Mesocarp lipase abundance correlates with lipase activity We devised a functional proteomic approach to identify lipases from a crude protein extract. The approach is based on the use of an inhibitor, tetrahydrolipstatin [22] , that can bind covalently to the lipase catalytic serine residue. Thus, a crude protein extract from ripe mesocarp from the HL genotype was incubated with radiolabelled tetrahydrolipstatin. A single protein band of 55 kDa was subsequently detected by autoradiography ( Fig. 3a ). De novo sequencing ( Supplementary Fig. S1A ) showed significant homology to a protein with high similarity to castor bean acid lipase [23] . The MS/MS spectra allowed us to identify from palm sequences [24] , [25] , [26] a cDNA named EgLIP1 (GenBank accession number JX556215 ), coding for a protein with strong homology to castor bean acid lipase (34.6% identity, 51.8% similarity, Supplementary Fig. S1 B ). Antibodies raised against a specific peptide detected a 55-kDa protein in HL mesocarp, whereas no protein could be detected in the mesocarp from the LL line ( Fig. 3b ). Immunolocalization data ( Fig. 3c ) showed that the putative lipase is localized adjacent to the outer surface of the lipid droplets. Taken together, these data suggest that EgLIP1 encodes the mesocarp lipase. 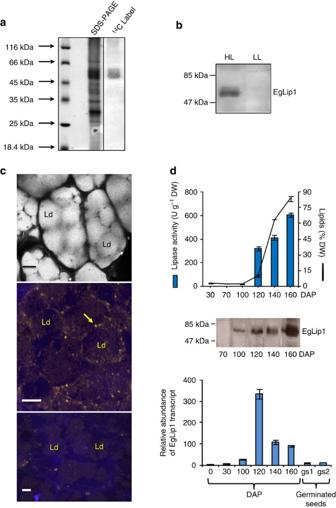Figure 3: Isolation and characterization of the oil palm mesocarp lipase EgLIP1. (a) Mesocarp crude protein extract was incubated with radioactive tetrahydrolipstatin and loaded on a 10% SDS-PAGE gel (left panel). The gel was dried and autoradiographed (right panel). (b) Western analysis of the EgLIP1 protein in the fruit mesocarp from LL and HL lines (D1 progenies). (c) Immunolocalization of EgLIP1. Confocal analysis of mesocarp sections stained with Nile red (upper panel) to detect lipids in lipid droplets (Ld)26labelled with anti-EgLIP1 and DAPI (middle panel) or pre-immune serum and DAPI as control (lower panel). Yellow arrow indicates anti-EgLIP1 signal (yellow spots) at border of Lds in mesocarp cell. Scale bar is 5 μm. (d) Lipase activity, lipid, EgLIP1 protein and transcript profiles in mesocarp during fruit ripening. Fruit and early germinated seedlings were from the P1 progeny. DAP: days after pollination. gs1, embryo from germinated seed; gs2, embryo from early post-germinated seed. Error bars represent s.d. Figure 3: Isolation and characterization of the oil palm mesocarp lipase EgLIP1. ( a ) Mesocarp crude protein extract was incubated with radioactive tetrahydrolipstatin and loaded on a 10% SDS-PAGE gel (left panel). The gel was dried and autoradiographed (right panel). ( b ) Western analysis of the EgLIP1 protein in the fruit mesocarp from LL and HL lines (D1 progenies). ( c ) Immunolocalization of EgLIP1. Confocal analysis of mesocarp sections stained with Nile red (upper panel) to detect lipids in lipid droplets (Ld) [26] labelled with anti-EgLIP1 and DAPI (middle panel) or pre-immune serum and DAPI as control (lower panel). Yellow arrow indicates anti-EgLIP1 signal (yellow spots) at border of Lds in mesocarp cell. Scale bar is 5 μm. ( d ) Lipase activity, lipid, EgLIP1 protein and transcript profiles in mesocarp during fruit ripening. Fruit and early germinated seedlings were from the P1 progeny. DAP: days after pollination. gs1, embryo from germinated seed; gs2, embryo from early post-germinated seed. Error bars represent s.d. Full size image To obtain more evidence for a role of EgLIP1 in the mesocarp, we studied its pattern of expression, protein accumulation and activity. Lipase activity assays revealed a >100-fold increase during the maturation and ripening stages [26] of fruit development ( Fig. 3d ), which coincided with the onset of lipid accumulation. The EgLIP1 transcript peak accumulation and the increase in the EgLIP1 protein ( Fig. 3d , Supplementary Fig. S2 ) occurred concomitant to lipase activity. Quantitative RT-PCR analysis of transcripts in select palm tissues indicated that the EgLIP1 gene is almost exclusively expressed in the mesocarp during fruit ripening. EgLIP1 transcript was not detected in the embryo, kernel, flowers, roots, leaves or the vegetative shoot apex ( Supplementary Fig. S3 ). In early post-germinated seedlings, the EgLIP1 transcript was present, but at 34-fold less than that observed in the mesocarp ( Fig. 3d , Supplementary Fig. S3 C ). To examine the relationships between EgLIP1 and the LL trait, lipase activity, transcript accumulation and the amounts of lipase protein were analyzed in the P2 segregating progeny ( Fig. 4a , Supplementary Fig. S2 , Supplementary Fig. S4 ). Low oil acidity was associated with LL activity, and barely detectable amounts of EgLIP1 protein and corresponding transcript, whereas high levels of acidity correlated with high levels of lipase activity, EgLIP1 protein and transcripts. These results provide strong evidence that oil acidity is directly related to the amount of transcript that encodes the EgLIP1 lipase. 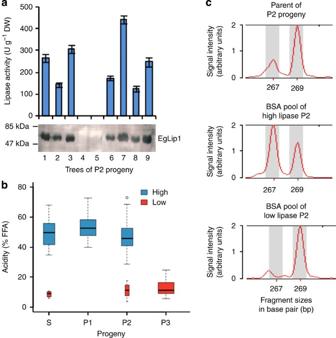Figure 4: The low-acidity trait is monogenic and cosegregates withEgLIP1lipase gene. (a) Lipase activity and EgLIP1 protein in P2 progeny. Error bars represent s.d. (b) Acidity measurements from the S, P1, P2 and P3 progenies. Selfing D1 led to a progeny of 21 trees (S), 3 of which were further self-crossed to give rise to progenies P1, P2 and P3 (see plant material in Material and Methods section). For each progeny, width of Boxplots is proportional to the number of trees per class. S and P2 showed a 3:1 ratio consistent with a monogenic recessive trait (S:χ2=0.016,P=0.90, d.f.=1; P2: χ2=0.205,P=0.65, d.f.=1) (c) The low-acidity trait is linked to theEgLIP1locus. The microsatellite marker EgCIR_LIP03 is located in the promoter region ofEgLIP1and shows two alleles that are visualized on electrophoregrams as 267 and 269-bp-long amplicons. Bulk segregation analysis was carried out on P2 progeny. Each genomic DNA pool (HL or LL) was represented by 10 randomly chosen trees in each acidity class. Figure 4: The low-acidity trait is monogenic and cosegregates with EgLIP1 lipase gene. ( a ) Lipase activity and EgLIP1 protein in P2 progeny. Error bars represent s.d. ( b ) Acidity measurements from the S, P1, P2 and P3 progenies. Selfing D1 led to a progeny of 21 trees (S), 3 of which were further self-crossed to give rise to progenies P1, P2 and P3 (see plant material in Material and Methods section). For each progeny, width of Boxplots is proportional to the number of trees per class. S and P2 showed a 3:1 ratio consistent with a monogenic recessive trait (S: χ 2 =0.016, P =0.90, d.f.=1; P2: χ 2 =0.205, P =0.65, d.f.=1) ( c ) The low-acidity trait is linked to the EgLIP1 locus. The microsatellite marker EgCIR_LIP03 is located in the promoter region of EgLIP1 and shows two alleles that are visualized on electrophoregrams as 267 and 269-bp-long amplicons. Bulk segregation analysis was carried out on P2 progeny. Each genomic DNA pool (HL or LL) was represented by 10 randomly chosen trees in each acidity class. Full size image The acidity trait cosegregates with mesocarp lipase gene To determine the inheritance of the low-acidity trait, we analyzed the D1 self-crossed progeny (S). Two groups were observed, one with an average FFA content of 11.6% and the other with 48.5% ( Fig. 4b ). The low-acidity group represented 23.8% of the progeny, which is consistent with a 3:1 Mendelian segregation and a recessive low-acidity trait. We further analyzed three progenies derived from two successive D1 self-crosses ( Fig. 4b ). One contained only HL individuals (P1), another only LL individuals (P3) and the third progeny (P2) showed a 3:1 segregation pattern similar to that of S. These results confirmed that the oil acidity trait is monogenic with the low acidity being recessive, and that D1 is indeed heterozygous for the trait. Notably, similar results were also obtained from D1 × L1 material ( Supplementary Fig. S5 ), which further indicated that the LL trait of D1 and L1 trees belonged to the same complementation group. Analysis of genomic DNA from S and P2 revealed the existence of a (TG) 8 (TA) 16 microsatellite marker locus ( mEgCIR_LIP03 ) between 744 bp and 792 bp upstream of the EgLIP1 initiating ATG codon, with two alleles that showed a few base differences. A bulk segregant analysis (BSA), carried out in the P2 progeny showed a cosegregation of mEgCIR_LIP03 with the oil acidity trait. Two marker alleles (267 bp and 269 bp) were present in the bulk for HL activity and one single marker allele (267 bp) in the bulk for LL activity ( Fig. 4c ). Our BSA with 10 genotypes per bulk showed a very low probability (2 × 10 −6 ) that this marker locus is polymorphic without a physical link with the major gene controlling the oil acidity. The cosegregation provides further evidence that EgLIP1 is the gene that controls oil acidity in the pulp of mature fruits, or is at least closely linked to another gene controlling the activity of EgLIP1 itself. In either case, the mEgCirLIP03 marker or EgLIP1 itself provide useful markers for introgression of the LL trait into other elite oil palm genotypes. Our results indicate the EgLIP1 transcript is almost exclusively present in the mesocarp, suggesting that EgLIP1 function is restricted to this tissue ( Supplementary Fig. S3 ). The oil contained in the mesocarp of oil palm fruit serves to attract disseminating animals and does not participate in the metabolism of other tissues and organs of the plant. One can speculate that the lipase function may enhance the palatability of fat, given this is due in part to receptors to fatty acids and not to triacylglycerol [27] , therefore increasing fruit attractiveness towards disseminating animals. As the main components of yield are not affected in LL trees ( Table 1 ), the LL allele was evidently not selected against by breeders. As Deli genotypes originated from a narrow (4 trees) genetic basis, the LL allele is likely present in a significant number of elite trees currently used for seed production. Indeed, a previous study allowed us to identify 4 LL trees out of 37 (ref. 11 ). We are currently screening a wide range of material for the LL allele to assess whether the microsatellite marker can be used in genotypes other than Deli and to increase our mapping population to achieve fine mapping of the trait. Preliminary mapping data confirm BSA results (N. Billotte, unpublished data). The availability of a molecular marker for the trait will allow breeders to rapidly identify potent genitors that carry a LL allele, and to introgress the trait into main elite genotypes during the next breeding cycle for seed production. The low-lipase genotypes should allow more flexibility in the management of harvest and bunch processing. Delaying harvest by 10 days in large estates should still reduce losses in the form of FFA, provide an additional 2–3% oil yield due to extended ripening and reduce harvesting frequency by one-third, thus lowering labour costs. Taken together, these impacts should represent an economic gain of ~1 billion dollars per year, based on today’s production. Substantially higher gains are anticipated provided the LL trait is associated to non- or low-shedding fruits [28] . However, the most important benefits are likely to be for African smallholders whose improved oil will gain access to international markets. Plant material All plant material were derived either from a cross between a tree (D1) from the Deli population and a tree (L1) from the La Me population or from progenies of D1 ( Supplementary Fig. S6 ). The offspring of D1 × L1 cross corresponds to elite material planted worldwide. This cross was used to assess the performances of LL trees, unless otherwise indicated. Analyses were conducted using progenies from D1. S progeny resulted from self-crossing of D1 and contains 21 trees, 5 of which were further self-crossed to give rise to progenies P1 (15 trees), P2 (104 trees), P3 (17 trees), P4 (75 trees) and P5 (75 trees). These trees are cultivated both at CRA-PP (Pobé, Bénin) and CEREPAH (La Dibamba, Cameroon). A bunch was considered to be ripe when one to five fruits detached. Each experiment was performed 3–5 times. Identification of LL and HL trees The amount of endogenous lipase was estimated by measuring the percentage of FFA released from a mesocarp homogenate for 1 hour after tissue disruption [10] . Only attached, undamaged fruits that showed no visual signs of fungal infestation were used. Mesocarp (10 g) was ground with mortar and pestle and stored at room temperature for 1 hour. The mixture was extracted with hexane (10 ml g −1 of pulp) and debris filtered away. Hexane was evaporated and the oil dried in a desiccator for 1 hour. Oil acidity was titrated with 0.1 N KOH according to standard procedures [11] . FFA content was calculated based on the molecular mass of palmitic acid. Oil extraction from bunches Oil was extracted using procedures similar to those used at mills. Bunches were subdivided into spikelets, which were boiled for 1–2 h; the fruits detached manually and the oil was extracted using a screw-press. After decantation, the oil was skimmed, dried, and its acidity was determined by titration. Data were Box–Cox transformed to achieve a normal distribution, ascertained by Anderson–Darling test. Analyses of variance were performed according to the general linear model. Multiple mean comparisons were made by Tukey’s test. Fungicide treatment After harvest, each bunch was divided; one half was sprayed with a fungicide solution of DITHANE M45 (mancozeb 80%) at 2 g l −1 and the other was used as a control, and sprayed with water. Both samples were sun-dried and kept in a closed room at room temperature for 6, 9 and 12 days before the oil was extracted. Multiple mean comparisons were made by Tukey’s test. Mesocarp constituent analyses For each stage of development, three independent bunches were collected from three individuals of the same progeny. Fifteen spikelets were collected in the centre of each bunch, from which five spikelets were randomly sampled. Three undamaged fruits were then randomly sampled from each of the five spikelets. Their mesocarp was dissected and flash-frozen in liquid nitrogen. Total lipids were extracted from 1-g samples of freeze-dried powder using a modified Folch method as described previously [29] . For all electrophoresis gel analyses, total mesocarp proteins were extracted using aqueous phenol [30] . Labelling the lipase with radioactive tetrahydrolipstatin was carried out as described [30] , except that THL was dissolved in hexane and added to the hexane extract of mesocarp without using detergent. The gel was dried and submitted to autoradiography. The labelled band was submitted to trypsin digestion and analyzed by LC-MS/MS at Bordeaux Proteomic Facility as described previously [30] , [31] . Lipase activity was assayed by continuous titration of released fatty acids with a pHSTAT [8] . Antibodies were raised by Biotem France against the peptides RDYVNGGRLAKITGKYS and DRKKGFPKELSRND. The peptides were conjugated to a protein carrier and injected with Freund complete adjuvant. Rabbits were boosted twice and exsanguinated at day 45. Total RNA from oil palm tissues was extracted as previously described [32] , [33] and 1 μg was used to synthesize cDNA using a first-strand cDNA synthesis kit (ImProm-II Reverse Transcription System, Promega). qPCR was conducted on a LightCycler 480 (Roche) in 96-well plates in a volume of 10 μl containing 2 μl of cDNA diluted 1/100, 1.5 μl of each primer (2 μM; 5′-ACTACGTCAACGGTGGAAGG-3′, 5′-CCGTTCCAAATCCAGTTCTT-3′) and 5 μl SYBR Green Mastermix (Roche). PCR was initiated by denaturation at 95 °C for 10 min, followed by 45 cycles of 95 °C for 15 s, 60 °C for 15 s and a final extension at 70 °C for 1 min. Transcript levels were normalized to that of EgEfα1 (GenBank accession number: AY550990 , oligonucleotides 5′-TATCAAAGGATGGGCAGACC-3′ and 5′-TCATCATACCTTGCCTTGGA-3′) mRNA, and relative mRNA abundance was determined as previously reported [34] . Control using RNA matrices were also conducted to validate the absence of DNA in each sample. Each time point was replicated three times from 3–5 independent biological samples, and all amplified cDNA fragments were sequenced by Beckman-Cogenics. Gene abundance is expressed as mean and standard error bars are calculated from three technical replicates. Immunolocalization of EgLIP1 lipase Mesocarp tissue samples were fixed in 0.1 M PBS buffer containing 8% ( w / v ) paraformaldehyde and 4% ( w / v ) N -(3-Dimethylaminopropyl)- N ′-ethylcarbodiimide hydrochloride for 16 h at 4 °C. Samples were subsequently washed in 0.1 M PBS buffer and cut into 150 μm sections using a vibratome. Sections were saturated in 0.1 M PBS containing 3% ( w / v ) foetal bovine serum for 24 h at 4 °C and transferred into 0.1 M PBS buffer containing either anti-EgLIP1 antibodies or pre-immune serum (diluted 1/100) for 24 h at 4 °C. Sections were then washed 4 times in 0.1 M PBS and transferred into a 0.1 M PBS solution containing goat anti-rabbit IgG antibody Alexa Fluor 545 conjugated (dilution 1/500) for 3 h. Sections were washed four times in PBS (0.1 M) and transferred to PBS buffer containing DAPI (14.3 μM) to visualize nucleus and membrane of oil droplets. Observation was performed using a confocal microscope (Zeiss LM510 meta) at magnifications × 40/1.2 numeric aperture, at the Cirad imagery facility (Montpellier, France). Excitation was performed at 543 nm for Alexa Fluor 545 and at 405 nm for DAPI. Cloning and sequencing of the EgLIP1 genomic region A bacterial artificial chromosome (BAC) library (92,160 clones, ~6 genome equivalents) made from the oil palm genotype L1 was screened using EgLIP1 cDNA as a probe. Three positive BAC clones were sequenced (with at least 50-fold coverage) using the Roche/454 GS FLX sequencing technique and assembled by Beckman-Cogenics (USA). The BAC contigs were assembled into one single haplotype sequence using CodonCodeAligner version 3.7.1 (CodonCode Corporation, USA), although the tree used as source of DNA proved to be heterozygous for the lipase trait. A search of microsatellite loci in the EgLIP1 genomic region and the design of PCR primers for microsatellite locus mEgCirLIP03 were performed using the SSR Analysis Tool (SAT) software [35] . Bulk segregant analysis Genomic DNA was extracted using the commercial kit NucleoSpin 96 Plant according to the manufacturer instructions (Macherey-Nagel, Germany). Legitimacy of P2 genotypes was confirmed by ADN id (Montpellier, France) company using 14 E. guineensis microsatellite markers [36] . A BSA was performed on the progeny P2 showing a 3:1 Mendelian segregation pattern for the oil acidity trait. The mEgCIR_LIP03 marker locus was amplified in the parent of P2 and in two equimolar mixtures of 10 DNAs each and made from P2 individuals randomly chosen within the two extreme phenotypic classes of oil acidity: (i) of HL phenotypes (oil acidity >40%) supposed to be homozygous (++) or heterozygous (+−) for EgLIP1 , and (ii) of LL genotypes (acidity <20%) supposed homozygous (−−) for that gene. The DNAs were PCR amplified in condition of fluorescence [36] , [37] using the mEgCirLIP03 primers (forward: 5′-TCAAAGAAACTTGTAGCATATATCAAA-3′; reverse: 5′-CATCCAGTAAGCTAACACACAAATG-3′) in a Mastercycler ep 384 thermocycler (Eppendorf, Germany) on 25 ng of DNA in a 10 μl final volume of buffer (10 mM Tris–HCl (pH 8), 200 μM of dNTP, 0.5 μM MgCl 2 , 0.05% w / v gelatin) containing 0.08 μM of the M13-labelled primer, 0.1 μM of the other primer and 1 U of Taq DNA polymerase. The PCR programme was: initial denaturation at 94 °C for 4 min; 10 «Touchdown» cycles each of 94 °C for 45 s, 55 °C (−0.5 °C per cycle) for 1 min, 72 °C for 1 min; and then 25 cycles of 94 °C for 45 s, 50 °C for 60 s and 72 °C for 60 s; and a final elongation step at 72 °C for 30 min. The PCR products were revealed by capillary electrophoresis on an Applied Biosystems 3500xL Genetic Analyzer (Life Technologies, USA) and the chromatogram allelic patterns were analyzed under the GeneMapper Software version 4.1 (Life Technologies, USA). Determination of yield components Ripe bunches were collected and analyzed as previously described [38] . Oil was extracted and quantified as described above. Results were analyzed using SAS v9.2 software (MIXED Procedure, SAS Institute, http://www.sas.com ): a one-way analysis of variance (factor group) was carried out and the model’s residuals were studied to test the model’s validity (normality, outliers). The tree/bunch effect was tested with a likelihood ratio test. If significant, it was kept in the model as a random effect. The results were expressed using a 95% confidence interval and a margin of error of 5%. How to cite this article: Morcillo, F. et al. Improving palm oil quality through identification and mapping of the lipase gene causing oil deterioration. Nat. Commun. 4:2160 doi: 10.1038/ncomms3160 (2013).